Arabidopsisubiquitin ligase MIEL1 mediates degradation of the transcription factor MYB30 weakening plant defence One of the most efficient plant resistance reactions to pathogen attack is the hypersensitive response, a form of programmed cell death at infection sites. The Arabidopsis transcription factor MYB30 is a positive regulator of hypersensitive cell death responses. Here we show that MIEL1 ( M YB30- I nteracting E 3 L igase 1 ), an Arabidopsis RING-type E3 ubiquitin ligase that interacts with and ubiquitinates MYB30, leads to MYB30 proteasomal degradation and downregulation of its transcriptional activity. In non-infected plants, MIEL1 attenuates cell death and defence through degradation of MYB30. Following bacterial inoculation, repression of MIEL1 expression removes this negative regulation allowing sufficient MYB30 accumulation in the inoculated zone to trigger the hypersensitive response and restrict pathogen growth. Our work underlines the important role played by ubiquitination to control the hypersensitive response and highlights the sophisticated fine-tuning of plant responses to pathogen attack. Overall, this work emphasizes the importance of protein modification by ubiquitination during the regulation of transcriptional responses to stress in eukaryotic cells. Plants do not have specialized immune cells but they have developed a complex cell-autonomous defence network to fight off invading pathogens. Defence activation in plants is frequently associated with the development of the so-called hypersensitive response (HR), a type of programmed cell death at the infection site that prevents the spread of the pathogen inside the plant [1] . The sharp boundary of the HR suggests the existence of efficient mechanisms that control cell death and survival. Nevertheless, the regulatory mechanisms of HR development and restriction remain largely unknown. Activation of immunity is achieved by multiple transcriptional regulators that reprogram cell transcription to favour defence over routine cellular requirements [2] . The arsenal of transcriptional regulators consists not only of DNA-binding transcription factors (TFs) but also of proteins that interact with and regulate these TFs. We previously identified MYB30, an Arabidopsis R2R3-type MYB TF, as a positive regulator of plant defence and HR responses. MYB30 activates genes related to the lipid biosynthesis pathway that leads to the production of very-long-chain fatty acids (VLCFAs [3] , [4] ). Interestingly, we recently showed that MYB30 is targeted by the Xanthomonas campestris pv. campestris ( Xcc ) effector XopD, suppressing MYB30 transcriptional activity and thereby plant resistance [5] . All these data underline MYB30 as an important regulator of plant defenses. Cellular signals that are perceived by TFs and that modulate their activity are diverse and include changes in cell redox status, calcium spiking and protein phosphorylation or ubiquitination [2] . Ubiquitination is a common post-translational modification that consists of covalent binding of ubiquitin (Ub) to lysine residues in target proteins. Ub is a signalling module for a variety of cellular processes, including DNA repair, gene transcription, protein activation or receptor trafficking, although the best-characterized function of Ub is associated to selective protein degradation through the 26S proteasome [6] . Ubiquitination involves an enzymatic cascade that implicates Ub-activating (E1), Ub-conjugating (E2) and Ub-ligase (E3) enzymes. E3 proteins are classified into four main subfamilies depending on their structure and mechanism of action: HECT ( H omologous to E 6-associated protein C - T erminus), RING ( R eally I nteresting N ew G ene), U-Box and cullin-RING ligases [6] . HECT proteins are unique because they form an Ub-E3 intermediate before transfer of Ub to the substrate [7] . RING and U-Box proteins are structurally related single polypeptides that respectively use zinc chelation and hydrogen bonds/salt bridges to transfer Ub from the Ub-E2 intermediate to the target [8] , [9] . E3 ligases containing a RING domain can act independently or as part of a multisubunit cullin-RING ligase complex such as SCF ( S kp1, C ullin, F -box-type ligase). In this complex, substrate recognition is provided by the F-box protein, whereas a RING protein binds to the E2. By contrast, some RING domain-containing E3 ligases act independently and determine substrate specificity allowing the interaction between the E2 and the target protein by tethering them in close proximity [6] , [10] . To better understand the regulation and mode of action of MYB30, we previously performed a yeast two-hybrid (Y2H) screen to search for MYB30 protein partners and identified a secretory phospholipase ( At sPLA 2 -α) that exerts negative spatial and temporal control on MYB30 transcriptional activity [11] . Here, we describe a new MYB30-interacting partner encoding a RING E3 Ub ligase protein that we named MIEL1 ( M YB30- I nteracting E 3 L igase 1 ). We demonstrate that MIEL1 is an active E3 ligase that interacts with MYB30 in the plant cell nucleus. Moreover, MIEL1 ubiquitinates MYB30 thereby leading to its degradation by the 26S proteasome. Arabidopsis miel1 mutant plants display enhanced HR and resistance after inoculation with avirulent bacteria. These phenotypes are MYB30-dependent and correlate with downregulation of MYB30 target gene expression. Finally, modulation of MIEL1 expression provides an efficient regulatory mechanism to (i) attenuate the activation of defence and related cell death responses in the absence of the pathogen and (ii) promote MYB30 accumulation and triggering of the HR/defence at the site of inoculation. In summary, this work underlines the importance of transcription regulation by ubiquitination during the establishment of plant defence reactions, which is a shared feature in eukaryotic cells in response to a variety of stress cues. Identification of MIEL1 In order to search for MYB30-interacting partners, a MYB30 version deleted from its C-terminal transcriptional activation domain (MYB30ΔAD) was previously used as bait to screen a Y2H Arabidopsis cDNA library generated from mRNAs isolated from leaf tissue inoculated with the strain 147 of Xcc [11] . Here we describe the identification of a cDNA clone encoding a non-characterized Zinc Finger RING-type protein (At5g18650) that we named MIEL1. RING domains are characterized by the presence of a cysteine-rich domain in which, similar to the zinc finger domain, Cys and/or His residues coordinate two zinc ions [8] . RING proteins are classified based on the nature of the metal ligand residues present in the RING domain and/or the number of amino acids between them. According to this classification, MIEL1 belongs to C3H2C3 canonical RING type (also called RING-H2), which presents Cys residues at metal ligand positions 1, 2 and 3, His residues at positions 4 and 5, and again Cys residues at positions 6, 7 and 8 ( Supplementary Fig. S1 ). RING domains have been shown to be essential for catalysing E3 Ub ligase activity [8] . Coexpression of full-length MIEL1 and MYB30ΔAD resulted in yeast growth on selective medium, whereas yeast cells expressing both MIEL1 and the unrelated MYB TF MYB123 (ref. 12 ) did not grow ( Supplementary Fig. S2 ). Furthermore, no protein interaction could be detected in yeast coexpressing MYB30ΔAD and an additional Zinc Finger RING C3H2C3-type protein that we called RINGc (RING control; At1g61620). Together, these data demonstrate the specificity of the interaction between MIEL1 and MYB30 in yeast. MYB30 and MIEL1 physically interact in the plant cell nucleus MYB30 was previously localized to the nucleus of Arabidopsis and N. benthamiana cells [11] . A MIEL1-YFPv fusion shows a homogenous distribution in the cytoplasm and nucleus of Arabidopsis cells ( Fig. 1 ). Moreover, the nuclear colocalization of MYB30-CFP and MIEL1-YFPv suggests a possible interaction between the two proteins in planta ( Fig. 1 ). This idea was investigated using FRET-FLIM assays. A significant reduction of the average CFP lifetime was measured in Arabidopsis nuclei coexpressing the MYB30-CFP and MIEL1-YFPv fusion proteins, as compared with nuclei expressing MYB30-CFP alone ( Fig. 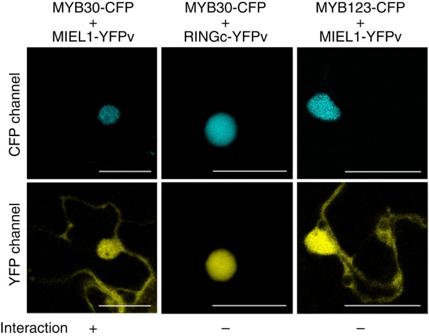Figure 1: MIEL1 colocalizes with MYB30 in the nucleus. Confocal images of epidermal cells of Arabidopsis seedlings 72 h afterAgrobacterium-mediated transient expression of the indicated constructs. The interaction (+) between MYB30 and RING proteins as determined by Y2H and FRET-FLIM is indicated. Bars, 15 μm. 1 ; Table 1 ), showing that MIEL1 is able to interact with MYB30 in the nucleus. Despite the nuclear colocalization between MYB30-CFP and RINGc-YFPv, no physical interaction could be detected between the two proteins, confirming the specificity of the MYB30/MIEL1 protein interaction ( Fig. 1 ; Table 1 ). Furthermore, no physical interaction could be detected between the nuclear localized TF MYB123-CFP [12] and MIEL1-YFPv ( Fig. 1 ; Table 1 ). The same results were obtained in N. benthamiana epidermal cells ( Supplementary Fig. S3 ; Supplementary Table S1 ). Taken together, our data demonstrate the specific physical interaction between MYB30 and MIEL1 in living plant cells. Figure 1: MIEL1 colocalizes with MYB30 in the nucleus. Confocal images of epidermal cells of Arabidopsis seedlings 72 h after Agrobacterium -mediated transient expression of the indicated constructs. The interaction (+) between MYB30 and RING proteins as determined by Y2H and FRET-FLIM is indicated. Bars, 15 μm. Full size image Table 1 FRET-FLIM analysis show that MYB30 physically interacts with MIEL1 in Arabidopsis cell nuclei. Full size table MIEL1 is an active E3 ligase able to ubiquitinate MYB30 in vitro To determine whether MIEL1 displays E3 Ub ligase activity, in vitro ubiquitination assays were performed using a commercial yeast E1 protein as well as a GST-tagged Arabidopsis E2 protein (UBC8) and His-tagged MIEL1 fusion proteins purified from Escherichia coli . As expected, the E2 protein was ubiquitinated in the presence of the E1 independently of MIEL1 ( Fig. 2 , lane 5). When MIEL1 was added to the reaction, a protein ladder was detected using anti-Ub antibodies ( Fig. 2 , lane 2). The observed E3 Ub ligase activity of MIEL1 was dependent on the presence of E1 and E2 ( Fig. 2 , lanes 7 and 8), and abolished by mutations in the catalytic RING domain in which key amino acids Cys172, H174 and H177 were mutated to Ala [8] (MIEL1m; Fig. 2 , lane 4). 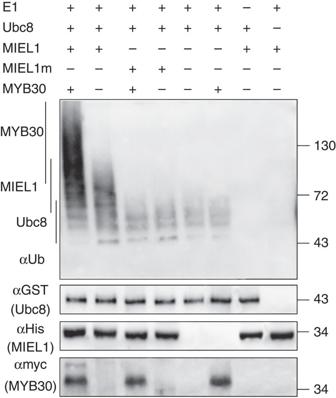Figure 2: MIEL1 is an active E3 ligase and ubiquitinates MYB30in vitro. His-tagged MIEL1 was tested for E3 Ub ligase activity in presence or absence of yeast E1, Arabidopsis E2 (UBC8) and MYB30. Anti-Ub, anti-GST, anti-His and anti-myc antibodies were used to detect ubiquitinated proteins, UBC8, MIEL1 and MYB30, respectively. An integral RING catalytic domain is required to detect MIEL1-mediated ubiquitination that is not observed when using MIEL1m. Molecular mass markers in kilodaltons are indicated on the right. Figure 2: MIEL1 is an active E3 ligase and ubiquitinates MYB30 in vitro . His-tagged MIEL1 was tested for E3 Ub ligase activity in presence or absence of yeast E1, Arabidopsis E2 (UBC8) and MYB30. Anti-Ub, anti-GST, anti-His and anti-myc antibodies were used to detect ubiquitinated proteins, UBC8, MIEL1 and MYB30, respectively. An integral RING catalytic domain is required to detect MIEL1-mediated ubiquitination that is not observed when using MIEL1m. Molecular mass markers in kilodaltons are indicated on the right. Full size image We next tested whether MYB30 is a substrate for MIEL1 E3 Ub ligase activity. Incubation of myc-tagged MYB30 with E1, UBC8 and MIEL1 led to the detection of a stronger and higher protein ladder than that corresponding to MIEL1 self-ubiquitination ( Fig. 2 , lane 1). Furthermore, a modified form of MYB30 was detected when using anti-myc antibodies, reflecting MYB30 post-translational modification by ubiquitination. Detection of the protein ladder and this modified MYB30 form were dependent on the presence of MIEL1 ( Fig. 2 , lane 6) and on the integrity of the RING catalytic domain, as they were not detectable after incubation with MIEL1m ( Fig. 2 , lane 3). Finally, an previously described active RING-type E3 ligase protein (At5g37270) [8] was not able to ubiquitinate MYB30 in vitro , further demonstrating the specificity of MIEL1-mediated ubiquitination of MYB30 ( Supplementary Fig. S4 ). Taken together, these results demonstrate that (i) MIEL1 is a functional E3 Ub ligase able to ubiquitinate MYB30 in vitro and that (ii) MIEL1 enzymatic activity depends on the structure of the RING domain. MYB30 is ubiquitinated by MIEL1 in planta To investigate whether MYB30 may be ubiquitinated in planta , we first tested whether MYB30 protein abundance is controlled by the plant 26S proteasome. Treatment with the proteasome inhibitor MG132 stabilized MYB30 expression in Arabidopsis transgenic plants overexpressing TAP-tagged MYB30 (ref. 11 ) (MYB30 OE ; Fig. 3a ). We next purified poly-ubiquitinated proteins from Col-0 wild-type and MYB30-TAP expressing Arabidopsis using a tandem Ub-binding entities (TUBEs) agarose resin. This resin specifically recognizes tetra-Ub and allows purification of poly-ubiquitinated proteins in native conditions [13] . In this assay, a smear corresponding to purified poly-ubiquinated proteins was detected using an anti-Ub antibody and, as expected, the detected signal was stronger in the presence of MG132 in both Col-0 and MYB30 OE plants ( Fig. 3b ). By contrast, when using an anti-TAP antibody, a protein ladder that was stronger in presence of MG132 was specifically detected in MYB30 OE Arabidopsis, whereas no signal was detected in Col-0 ( Fig. 3b ). No signal was detected when using uncoupled agarose beads either with anti-Ub or anti-TAP antibodies, demonstrating the specificity of binding of poly-ubiquitinated proteins to the TUBEs resin. Together, these results show that MYB30 is ubiquitinated in Arabidopsis. 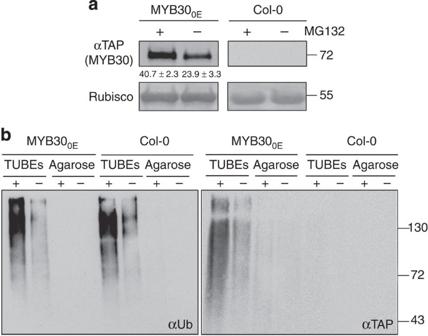Figure 3: MYB30 is ubiquitinated inArabidopsis. (a) Arabidopsis wild-type Col-0 and transgenic plants overexpressing TAP-tagged MYB30 (MYB30OE) were treated with the proteasome inhibitor MG132 (+) or the solvent DMSO (−). Mean and s.e.m. densitometry values for MYB30-TAP were calculated from six independent experiments. (b) Following MG132 treatment, ubiquitinated proteins were purified using the TUBEs resin. Agarose resin was used to detect non-specific protein binding. Western blot with anti-Ub and anti-TAP antibodies detects ubiquitinated proteins and TAP-tagged MYB30, respectively. Ponceau S staining confirms equal loading. Molecular mass markers in kilodaltons are indicated on the right. Figure 3: MYB30 is ubiquitinated in Arabidopsis . ( a ) Arabidopsis wild-type Col-0 and transgenic plants overexpressing TAP-tagged MYB30 (MYB30 OE ) were treated with the proteasome inhibitor MG132 (+) or the solvent DMSO (−). Mean and s.e.m. densitometry values for MYB30-TAP were calculated from six independent experiments. ( b ) Following MG132 treatment, ubiquitinated proteins were purified using the TUBEs resin. Agarose resin was used to detect non-specific protein binding. Western blot with anti-Ub and anti-TAP antibodies detects ubiquitinated proteins and TAP-tagged MYB30, respectively. Ponceau S staining confirms equal loading. Molecular mass markers in kilodaltons are indicated on the right. Full size image To test whether MYB30 ubiquitination in planta may be mediated by MIEL1, we used transient assays in N. benthamiana . As in Arabidopsis, MYB30 protein level was stabilized in N. benthamiana leaves transiently expressing FLAG-tagged MYB30 after treatment with the proteasome inhibitor MG132, whereas no effect on the accumulation of the control GUS protein was detected in the same conditions ( Supplementary Fig. S5 ). As MIEL1 is able to ubiquitinate MYB30 in vitro, we next investigated whether MYB30 proteasomal degradation may be induced by its interaction with MIEL1 in planta . Indeed, MYB30 protein accumulation was reduced when transiently coexpressed with MIEL1 in N. benthamiana ( Fig. 4a ). Importantly, MG132 treatment protected MYB30 from degradation, confirming that MIEL1-mediated degradation of MYB30 is proteasome dependent. In addition, the MIEL1 catalytic mutant MIEL1m that is unable to ubiquitinate MYB30 in vitro was used. Although mutations in MIEL1m did not modify the subcellular localization of the protein ( Supplementary Fig. S3 ) or its ability to interact with MYB30 ( Supplementary Table S1 ), coexpression with MIEL1m did not affect MYB30 protein accumulation, demonstrating that the catalytic activity of MIEL1 is required to negatively regulate MYB30 protein levels ( Fig. 4a ). Finally, MIEL1 expression did not modify protein accumulation of MYB123, consistent with the lack of physical interaction between the two proteins ( Fig. 4a ; Supplementary Table S1 ). 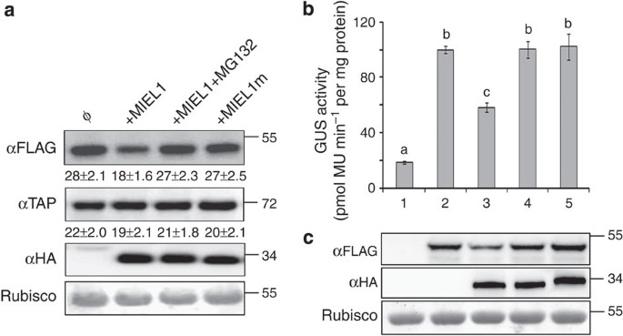Figure 4: MIEL1 leads to MYB30 proteasomal degradation and repression of its transcriptional activity. (a) FLAG-tagged MYB30 or TAP-tagged MYB123 were expressed inN. benthamianaalone or with haemagglutinin (HA)-tagged MIEL1 or MIEL1m, and treated or not with the proteasome inhibitor MG132, as indicated. Western blot analysis shows the expression of FLAG-tagged MYB30, TAP-tagged MYB123 and HA-tagged MIEL1 proteins. Mean and s.e.m. densitometry values for MYB30-FLAG and MYB123-TAP were calculated from six independent experiments and are shown at the bottom of each western blot. Ponceau S staining confirms equal loading. Molecular mass markers in kilodaltons are indicated on the right. (b) Fluorimetric GUS assays in leaf discs 36 hpi of the following constructs: (1)KCS1p:GUS reporter alone or with (2) MYB30-FLAG; (3)MYB30-FLAG+MIEL1-HA; (4) MYB30-FLAG+MIEL1m-HA; and (5) MYB30-FLAG+RINGc-HA. Statistical significance according to a Student’st-testP-value <10−5is indicated by letters. MU, methylumbelliferone. (c) Western blot showing expression of MYB30-FLAG and HA-tagged RING-type protein constructs. Ponceau S staining confirms equal loading. Molecular mass markers in kilodaltons are indicated on the right. Figure 4: MIEL1 leads to MYB30 proteasomal degradation and repression of its transcriptional activity. ( a ) FLAG-tagged MYB30 or TAP-tagged MYB123 were expressed in N. benthamiana alone or with haemagglutinin (HA)-tagged MIEL1 or MIEL1m, and treated or not with the proteasome inhibitor MG132, as indicated. Western blot analysis shows the expression of FLAG-tagged MYB30, TAP-tagged MYB123 and HA-tagged MIEL1 proteins. Mean and s.e.m. densitometry values for MYB30-FLAG and MYB123-TAP were calculated from six independent experiments and are shown at the bottom of each western blot. Ponceau S staining confirms equal loading. Molecular mass markers in kilodaltons are indicated on the right. ( b ) Fluorimetric GUS assays in leaf discs 36 hpi of the following constructs: (1) KCS1p: GUS reporter alone or with (2) MYB30-FLAG; (3)MYB30-FLAG+MIEL1-HA; (4) MYB30-FLAG+MIEL1m-HA; and (5) MYB30-FLAG+RINGc-HA. Statistical significance according to a Student’s t -test P -value <10 −5 is indicated by letters. MU, methylumbelliferone. ( c ) Western blot showing expression of MYB30-FLAG and HA-tagged RING-type protein constructs. Ponceau S staining confirms equal loading. Molecular mass markers in kilodaltons are indicated on the right. Full size image MIEL1 negatively regulates MYB30 transcriptional activity in N. benthamiana MYB30 promotes activation of the promoter of the KCS1 gene ( KCS1p ), involved in the biosynthesis of VLCFAs [4] . To study the functional role of the interaction between MYB30 and MIEL1, the effect of MIEL1 on MYB30-mediated transcriptional activation of KCS1p fused to the GUS reporter gene was tested in N. benthamiana . Consistent with previous results [4] , overexpression of MYB30 induced KCS1p transcriptional activation ( Fig. 4b , lane 2). In agreement with MYB30 reduced protein accumulation, MYB30-TAP-mediated transcriptional activation of KCS1p was significantly reduced when coexpressed with MIEL1 ( Fig. 4b ; lane 3). By contrast, no effect on KCS1p activation or MYB30 protein accumulation was observed when RINGc was coexpressed with MYB30 ( Fig. 4b , lane 5), indicating the specificity of the effect of MIEL1 in the control of MYB30 transcriptional activity. Finally, when coexpressed with MIEL1m, MYB30 protein accumulation and transcriptional activation of KCS1p were not affected ( Fig. 4b ; lane 4), confirming that MIEL1-mediated suppression of MYB30 accumulation and transcriptional activity require an intact RING domain in MIEL1. MIEL1 attenuates MYB30-mediated responses to bacterial infection To investigate the function of MIEL1 in the plant response to bacterial inoculation, we used an Arabidopsis miel1 knockout line from the SALK collection ( http://signal.salk.edu ) containing a T-DNA insertion at position +567 of the predicted open reading frame (SALK_097638 line; Supplementary Fig. S6A ). Absence of MIEL1 transcripts in homozygous miel1 knockout plants was confirmed by semiquantitative RT-PCR using MIEL1 gene-specific primers ( Supplementary Fig. S6B ). Similar to MYB30 OE plants, miel1 mutant plants showed clear HR cell death symptoms 64 hpi with Pseudomonas syringae pv. tomato DC3000 expressing the avirulence gene AvrRpm1 (Pst AvRpm1) , whereas Col-0 wild-type plants only showed chlorosis symptoms at this time ( Fig. 5a ). This phenotype was quantified by ion leakage measurements in leaf disk assays. Indeed, conductivity values measured in miel1 and MYB30 OE plants were higher than those displayed by Col-0 plants after bacterial inoculation ( Fig. 5b ). In agreement with faster HR development, miel1 plants showed increased resistance in response to inoculation with Pst AvrRpm1 and Pst AvrPphB , as compared with wild-type plants ( Fig. 5c , Supplementary Fig. S7 ), confirming the role of MIEL1 as a negative regulator of plant defence. Importantly, the increased HR and resistance phenotype displayed by the miel1 mutant was suppressed in a myb30 mutant background ( miel1/myb30 ; Fig. 5b ), demonstrating that the negative regulation of defence responses by MIEL1 is achieved via its effect on MYB30. 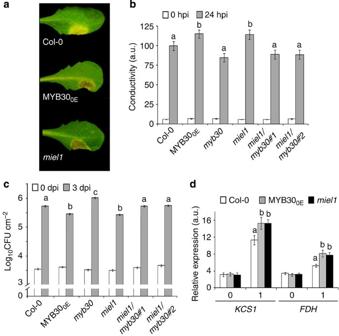Figure 5: MIEL1 is a negative regulator of resistance and HR responses inArabidopsisin response to bacterial inoculation. (a) Symptoms developed by the indicated Arabidopsis lines 64 hpi withPst AvrRpm1(2 × 106cfu ml−1). Pictures are representative of three independent experiments in which five plants of each line were infiltrated. (b) Quantification of cell death by measuring electrolyte leakage before (white bars) and 24 h after inoculation (grey bars) of the indicated lines withPst AvrRpm1(5 × 106cfu ml−1). Cell death values are related to the value displayed by wild-type Col-0 plants, which is set at 100%. Statistical differences using multiple factor analysis of variance (ANOVA) (P<10−4) are indicated by letters. (c) Growth ofPst AvrRpm1in the indicated Arabidopsis lines. Bacterial growth 0 (white bars) and 3 days (grey bars) was measured after inoculation (5 × 105cfu ml−1). Mean bacterial densities were calculated from six independent experiments with six individual plants (four leaves per plant). Statistical differences according to a Multiple Factor ANOVA test (P<0.01) are indicated by letters. (d) Expression analysis of the MYB30 target genesKCS1andFDHin the indicated Arabidopsis lines after inoculation withPst AvrRpm1(5 × 107cfu ml−1). Expression values of the individual genes were normalized usingSANDfamily andβ-tubulin4as internal standards. Statistical differences according to a Student’st-testP-value <0.05 are indicated by letters. 0 and 1 indicate hours postinoculation. Figure 5: MIEL1 is a negative regulator of resistance and HR responses in Arabidopsis in response to bacterial inoculation. ( a ) Symptoms developed by the indicated Arabidopsis lines 64 hpi with Pst AvrRpm1 (2 × 10 6 cfu ml −1 ). Pictures are representative of three independent experiments in which five plants of each line were infiltrated. ( b ) Quantification of cell death by measuring electrolyte leakage before (white bars) and 24 h after inoculation (grey bars) of the indicated lines with Pst AvrRpm1 (5 × 10 6 cfu ml −1 ). Cell death values are related to the value displayed by wild-type Col-0 plants, which is set at 100%. Statistical differences using multiple factor analysis of variance (ANOVA) ( P <10 −4 ) are indicated by letters. ( c ) Growth of Pst AvrRpm1 in the indicated Arabidopsis lines. Bacterial growth 0 (white bars) and 3 days (grey bars) was measured after inoculation (5 × 10 5 cfu ml −1 ). Mean bacterial densities were calculated from six independent experiments with six individual plants (four leaves per plant). Statistical differences according to a Multiple Factor ANOVA test ( P <0.01) are indicated by letters. ( d ) Expression analysis of the MYB30 target genes KCS1 and FDH in the indicated Arabidopsis lines after inoculation with Pst AvrRpm1 (5 × 10 7 cfu ml −1 ). Expression values of the individual genes were normalized using SAND family and β-tubulin4 as internal standards. Statistical differences according to a Student’s t -test P -value <0.05 are indicated by letters. 0 and 1 indicate hours postinoculation. Full size image Genetic complementation of the miel1 mutant was performed using a genomic MIEL1 construct (g MIEL1 ). Three independent homozygous g MIEL1 complemented T3 lines containing a single insertion of the wild-type MIEL1 gene were selected and inoculated with Pst AvrRpm1 . miel1 mutant plants containing the gMIEL1 construct displayed cell death and bacterial growth rates similar to those of wild-type Col-0 plants ( Supplementary Fig. S6 ), demonstrating that miel1 mutant phenotypes are causally related to the loss of function of MIEL1. Finally, as MYB30 OE plants, the miel1 null mutant line displayed higher expression of MYB30 VLCFA-related target genes, KCS1 and FDH, as compared with Col-0 wild-type plants following bacterial inoculation ( Fig. 5d ). These data confirm that MIEL1 negatively regulates Arabidopsis defence through repression of MYB30 transcriptional activity. MIEL1 and MYB30 expression are temporally and spatially regulated To gain further knowledge on the mode of action of MIEL1, wild-type Col-0 plants were inoculated with Pst AvrRpm1 and leaf samples harvested from areas both inside and immediately neighbouring the infiltrated zone at different times after inoculation. No significant modification of MYB30 or MIEL1 expression was observed in the area immediately neighbouring the inoculated zone ( Fig. 6 ). By contrast, in the inoculated zone, MYB30 expression was specifically induced 4 hpi, whereas MIEL1 expression was repressed after inoculation ( Fig. 6 ). Considering the negative control exerted by MIEL1 on MYB30 activity, these data indicate that MIEL1 contributes to the necessary attenuation of the plant defence response in the absence of the pathogen to avoid superfluous activation of defenses. Repression of MIEL1 expression after inoculation would remove this negative regulation and allow sufficient MYB30 accumulation in the infiltrated zone to trigger the development of the HR. 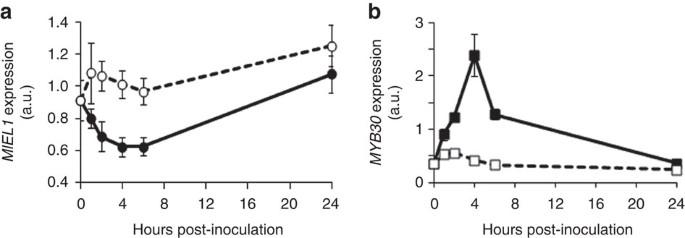Figure 6:MYB30andMIEL1gene expression is spatially and temporally regulated. Col-0 plants were inoculated withPst AvrRpm1(5 × 107cfu ml−1). Leaf samples were harvested from areas both inside and immediately neighbouring the infiltrated zone at the indicated time points. Relative expression ofMIEL1(a) andMYB30(b) in the inoculated (solid line) or in the adjacent (dashed line) zone was determined by Q-RT-PCR. Expression values were normalized usingSANDfamily andβ-tubulin4genes as internal standards. Mean and s.e.m. values were calculated from three experiments with three replicates. Figure 6: MYB30 and MIEL1 gene expression is spatially and temporally regulated. Col-0 plants were inoculated with Pst AvrRpm1 (5 × 10 7 cfu ml −1 ). Leaf samples were harvested from areas both inside and immediately neighbouring the infiltrated zone at the indicated time points. Relative expression of MIEL1 ( a ) and MYB30 ( b ) in the inoculated (solid line) or in the adjacent (dashed line) zone was determined by Q-RT-PCR. Expression values were normalized using SAND family and β-tubulin4 genes as internal standards. Mean and s.e.m. values were calculated from three experiments with three replicates. Full size image The Arabidopsis TF MYB30 is a positive regulator of Arabidopsis HR and defence responses. In this work we describe MIEL1, a previously uncharacterized Arabidopsis E3 Ub ligase, that contributes to the fine-tuning of plant defenses through ubiquitination and proteasomal degradation of MYB30. MIEL1 was identified in a Y2H screen of a cDNA library prepared from Arabidopsis leaves inoculated with avirulent bacteria using MYB30 as bait. In agreement with this finding, we have shown that MIEL1 and MYB30 colocalize and specifically interact in the plant cell nucleus. In addition, the fact that MIEL1 is able to ubiquitinate MYB30 in vitro provides further confirmation of this protein interaction. In an attempt to determine whether a particular region in MIEL1 is responsible for the interaction with MYB30, a series of YFP-tagged MIEL1 deletion N-terminal and C-terminal mutant proteins was engineered and the interaction of all these proteins with MYB30 was analysed using FRET-FLIM assays. As shown in Supplementary Table S1 , all MIEL1 deletions were unable to interact with MYB30 despite their subcellular localization and expression levels being undistinguishable from those of the full-length MIEL1 protein ( Supplementary Fig. S8 ). This finding suggests that the entire MIEL1 protein is required for its interaction with MYB30. Importantly, MIEL1 expression correlates with reduced MYB30 protein accumulation in planta . Moreover, the total number of N. benthamiana and Arabidopsis nuclei expressing MYB30-CFP is significantly reduced in the presence of MIEL1-YFPv, which rendered FRET-FLIM experiments a challenging task. Functional characterization of MIEL1 showed that this protein is an active E3 ligase able to ubiquitinate MYB30 and that, as previously described for other RING proteins, this activity depends on the integrity of key amino acids in the RING domain, which are essential for E2-dependent protein ubiqutination [8] . Finally, all these findings strongly suggest that epitope-tagging of the proteins does not affect their function. Approximately 6% of the Arabidopsis proteome is predicted to be involved in the Ub/proteasome system (UPS). Consistent with this prediction, the UPS has been implicated in the regulation of almost all aspects of plant growth and development, as well as in protection against biotic and abiotic stress [6] . In Arabidopsis, 1415 putative E3 ligases have been identified that are expected to allow the interaction between E2 enzymes and target proteins and, among them, 499 RING-type proteins have been predicted [10] . A significant number of UPS-related components, in particular E3 ligases, have been described as being involved in the regulation of plant immunity at all stages from pathogen recognition to downstream signalling, including hormone signalling pathways that regulate plant immune responses [14] , [15] , [16] . For example, following perception of bacterial flagellin, the Arabidopsis U-Box proteins PUB12 and PUB13 associate with the immune receptor FLS2, mediating its ubiquitination and degradation and providing an efficient mechanism of attenuation of basal defenses [17] . In addition, the Arabidopsis F-box protein CPR1 targets several resistance proteins for degradation, thereby regulating their accumulation and preventing autoimmunity [18] , [19] . The rice XA21-binding protein3 (XB3) is an active RING-type E3 ligase that binds to the kinase domain of the resistance protein XA21 and is substrate for the XA21 kinase activity [20] . Although XB3 is necessary for full accumulation of XA21 and for XA21-mediated resistance in rice, its targets remain to be discovered [20] . The important role of ubiquitination-related processes during the regulation of plant responses to pathogens is underlined by the finding that most microbes appear to have evolved a way to subvert the host UPS to promote disease [14] , [15] . Ubiquitination has a central role in different aspects of transcriptional regulation in animal cells, including (i) chromatin remodelling via histone modification and (ii) coordination of transcription initiation and elongation via ubiquitination of TFs and RNA polymerase II [21] . Here we show that MIEL1 E3 ligase activity targets the Arabidopsis MYB TF MYB30, providing a direct link between the MIEL1-mediated proteasomal degradation of MYB30, the negative regulation of MYB30 transcriptional activity and the suppression of Arabidopsis defence and HR responses. Moreover, the phenotypes associated to the miel1 mutation are lost in a myb30 mutant background, showing that the negative control exerted by MIEL1 on the establishment of defence is directly related to its action on MYB30. Interestingly, the intermediate resistance response displayed by miel1/myb30 plants, as compared with myb30 and miel1 plants, suggest the existence of additional defence-related MIEL1 targets that are functionally redundant with MYB30 during the regulation of Arabidopsis defence to pathogens. Although modulation of the expression of several RING genes in plants after treatment with different elicitors has been described [22] , [23] , [24] , [25] , only a few RING proteins have been involved in the regulation of plant immunity and, in most cases, their targets remain unknown. Moreover, the regulation by ubiquitination of the transcriptional activation related to disease resistance is yet poorly documented in plants. In Arabidopsis, the MYB TF BOS1 is required for resistance to several pathogens [26] . The RING-type E3 ligase BOI1 interacts with BOS1 in the plant cell nucleus and is able to ubiquitinate BOS1 in vitro, suggesting that BOS1 may be a target of BOI1 [27] . However, both bos1 mutant and BOI1 RNAi Arabidopsis plants, in which the BOS1 protein is expected to accumulate, display enhanced susceptibility to fungal infection. Therefore, whether BOI1 is able to directly regulate BOS1 protein accumulation remains unclear and no effect of BOI1 on BOS1 transcriptional activity has been reported [27] . In summary, our finding that MIEL1 regulates defence-related MYB30 transcriptional activation (i) highlights the crucial role played by ubiquitination in the transcriptional control of plant defence responses and (ii) provides a first description of a RING E3 Ub ligase that directly controls the transcriptional activation of the cell death associated to plant disease resistance. The importance of MYB30 as a regulator of resistance and associated HR responses to pathogen attack is highlighted by the recent finding that the type III Xcc effector XopD targets MYB30 in the plant cell nucleus to suppress its transcriptional activation and thereby plant defenses [5] . Interestingly, MYB30 activity is regulated not only by bacteria but also by plant cells. Indeed, we previously showed that, in the presence of MYB30, targeting of the secreted phospholipase At sPLA 2 -α is partially modified from Golgi-associated vesicles to the nucleus, where the two proteins interact, leading to repression of MYB30-mediated HR and defenses [11] . In this work, we report on the identification of MIEL1, a RING-type E3 Ub ligase that targets MYB30 for proteasomal degradation, negatively regulating transcriptional responses associated to the establishment of cell death. Data presented here, together with our previous work on At sPLA 2 -α, are consistent with the idea that At sPLA 2 -α and MIEL1 have essential, sequential and nonredundant roles in the regulation of MYB30 ( Supplementary Fig. S9 ). Indeed, MYB30 expression is specifically induced in the inoculated zone 4 hpi, whereas AtsPLA 2 -α expression peaks 6 hpi in the area immediately neighbouring the inoculated zone, suggesting that At sPLA 2 -α contributes to restrict the HR to the inoculated zone, thereby preventing spreading of cell death throughout the leaf [11] . MIEL1 expression is specifically inhibited after inoculation within the infiltrated zone, indicating that MIEL1 negatively regulates plant HR and defence activation through degradation of the MYB30 protein in the absence of the pathogen. After inoculation, repression of MIEL1 expression would remove this negative regulation and allow sufficient MYB30 accumulation to trigger HR and restrict pathogen growth. Finally, as MIEL1 expression remains constant in the adjacent zone, it is also possible that MIEL1-mediated degradation of MYB30 in this area may additionally contribute to avoid spreading of the HR beyond the inoculated zone. Considering these observations, Supplementary Fig. S9 illustrates our current working model for the regulation of MYB30-mediated HR responses. The fact that miel1 mutant plants do not show spreading HR after pathogen challenge suggests that additional factors ( At sPLA 2 -α and likely other regulators) control restriction of the HR to the inoculated zone. This hypothesis should be investigated in the future. In animal cells, the TFs p53 and c-Myc are central regulators of many key processes, including apoptosis. p53 and c-Myc represent excellent paradigms that illustrate the sophistication of transcription regulation by different post-translational modifications [28] , [29] . In particular, ubiquitination of these TFs provides efficient regulation of their stability, subcellular localization and activity [21] , [29] . In the case of c-Myc, a model has been proposed that suggests that Ub-mediated modulation of its transcriptional activity ensures tight control of highly active c-Myc that is potentially toxic to cells, for instance by inducing apoptosis [29] . Likewise, we propose that control of MYB30 transcriptional activity by ubiquitination contributes to the regulation of plant cell death responses associated to defence. Indeed, the establishment of defence is a costly response, closely connected to plant developmental processes, that requires a tight control to avoid deleterious effects to the host, as illustrated by HR lesion-mimic mutants that often present stunted growth and low fertility [1] , [30] . The existence of separate, nonredundant, negative regulatory mechanisms to control the HR thus provides an efficient means to temporally and spatially regulate the activation of programmed cell death and illustrates the sophisticated fine-tuning of plant responses to pathogen attack. Yeast assays The Y2H screen and methods used for identification of MIEL1 were previously described [11] . Briefly, an Arabidopsis thaliana Gal4 yeast two-hybrid cDNA prey library (MatchMaker; Clontech) was generated from mRNA isolated from leaves of 4-week-old plants (Ws-4 ecotype), syringe-infiltrated with the Xanthomonas campestris pv campestris 147 strain [4] . An AtMYB30 version deleted from its C-terminal activation domain (amino acids 1–234) was used as bait for screening 2 × 10 6 independent transformants exhibiting His auxotrophy on selective plates. Constructs Details of cloning procedures are provided as Supplementary Information . Plant and bacterial materials Arabidopsis lines used in this study were in the Columbia background and grown in Jiffy pots under controlled conditions in a growth chamber at 21 °C, with a 9-h light period and a light intensity of 190 μmol m −2 s −1 . The MYB30 ko line (GABIKAT T-DNA line 022F04) was reported before [31] . For transient expression of proteins in N. benthamiana, overnight bacterial cultures of Agrobacterium tumefaciens strain C58C1 expressing the protein of interest were harvested by centrifugation. Cells were resuspended in induction buffer (10 mM MgCl 2 , 10 mM Mes, pH 5.6, and 150 μM acetosyringone) to an OD 600 of 0.5. After 2 h at 22 °C, cells were infiltrated into leaves of 4-week-old N. benthamiana plants. Two days after A. tumefaciens infiltration, leaf discs used for experiments were harvested and processed, or frozen immediately in liquid nitrogen and stored at –80 °C. Transient expression of proteins in Arabidopsis seedlings was performed as described [32] . Briefly, A. tumefaciens overnight cultures were collected and resuspended at an OD 600 of 1 in 2 ml of 5% sucrose, 200 μM acetosyringone. Infiltration was performed by covering the seedlings with the Agrobacterium solution and by applying vacuum (10 mm Hg) twice for 1 min. Excess infiltration medium was subsequently removed and the plates transferred to a culture room for 3 days. Arabidopsis 4-week-old plants were kept at high humidity 12 h before inoculation and injected with a bacterial suspension of Pst A vrRpm1 or Pst Avr PphB at the indicated bacterial densities using a blunt syringe on the abaxial side of the leaves. For determination of in planta bacterial growth, leaves samples were harvested 0 and 3 days postinoculation and ground on sterile water. A predetermined dilution for each sample was plated on King’s B medium and incubated at 28 °C for 2 days. Data were submitted to a statistical analysis using Statgraphics Centurion XV.II Professional Software (Statpoint Technologies Inc., Warrenton, VA, USA). Normality of residues was verified by the Kolmogorov-Smirmov test. The effect of the genotype was tested by multiple factor analysis of variance. For proteaseome inhibition assays, 100 μM MG132 (Sigma-Aldrich) or the solvent DMSO (control) was infiltrated in N. benthamiana 24 h after agroinfiltration. Leaves were harvested 12 h after treatment. In Arabidopsis, 10-day-old seedlings were vacuum-infiltrated for 2 min with MG132 or DMSO and incubated for 4 h before harvesting. Fluorescence microscopy CFP and YFPv fluorescence was analysed with a confocal laser scanning microscope (TCS SP2-SE; Leica) using a × 63 water immersion objective lens (numerical aperture 1.20; PL APO). CFP fluorescence was excited with the 458 nm ray line of the argon laser and recorded in one of the confocal channels in the 465–520 nm emission range. YFP fluorescence was excited with the 514-nm line ray of the argon laser and detected in the range between 520 and 575 nm. Images were acquired in the sequential mode (20 Z plains per stack of images; 0.5 μm per Z plain) using Leica LCS software (version 2.61). FRET-FLIM Fluorescence lifetime of the donor was experimentally measured in the presence and absence of the acceptor. FRET efficiency ( E ) was calculated by comparing the lifetime of the donor in the presence ( τ DA ) or absence ( τ D ) of the acceptor: E =1−( τ DA )/( τ D ). Statistical comparisons between control (donor) and assay (donor+acceptor) lifetime values were performed by Student t -test. FRET-FLIM measurements were performed using a FLIM system coupled to a streak camera. The light source ( λ =439 nm) was a pulsed diode laser working at 2 MHz (Hamamatsu Photonics, Japan). All images were acquired with a × 60 oil immersion lens (Plan Apo 1.4 numerical aperture, IR) mounted on an inverted microscope (Eclipse TE2000E, Nikon, Japan) coupled to the FLIM system. The fluorescence emission was directed back out into the detection unit through a band pass filter. The FLIM unit was composed of a streak camera (Streakscope C4334, Hamamatsu Photonics, Japan) coupled to a fast and high sensitivity CCD camera (model C8800-53C, Hamamatsu). For each nucleus, average fluorescence decay profiles were plotted and lifetimes were estimated by fitting data with tri-exponential function using a non-linear least-squares estimation procedure. Recombinant protein purification and in vitro ubiquitination assays GST-UBC8, MYB30-myc, MIEL1-6His and MIEL1m-6His proteins were overexpressed and purified from E. coli Rosetta cell cultures using standard protocols. For in vitro ubiquitination assays reaction mixtures (20 μl) contained 0.5 μg of yeast ( Saccharomyces cerevisiae ) E1 enzyme (Sigma-Aldrich), 0.5 μg of purified Arabidopsis E2 enzyme UBC8, 0.5 μg of purified His-tagged MIEL1 protein as the E3 Ub ligase, and 1 μg of ubiquitin (Sigma-Aldrich) in 25 mM Tris-HCl, pH 7.5, 1 mM MgCl 2 , 1 mM ATP and 0.5 mM DTT. Reactions were incubated at 30 °C for 2 h and stopped by adding Laemmli buffer and boiling for 10 min. TUBEs pull down Protein extracts were prepared in 50 mM Tris-HCl, pH 7.4, 150 mM NaCl, 10% (v/v) glycerol, 1 mM PMSF, and 1% plant protease inhibitor cocktail (Sigma-Aldrich) and centrifuged at 14,000 g for 10 min at 4 °C. Protein concentration in the supernatant was determined with the Bradford protein assay kit (Bio-Rad) using BSA as a standard. For Ub immunoprecipitation assays, the deubiquitination inhibitor PR-619 (Tebu-bio) was added into the extraction buffer. Supernatants were pre-cleared for 30 min at 4 °C with agarose beads (Tebu-bio). Samples were split into two fresh tubes and used either for TUBEs (Tandem Ub-Binding Entities, Tebu-bio) or agarose beads (control) pull downs. All steps were performed at 4 °C. Pull downed proteins were eluted by boiling for 10 min in Laemmli buffer. Gel blot analysis Antibodies used for western blotting were anti-PAP soluble complex-HRP (Sigma, 1:2,000), anti-HA-HRP (3F10, Roche, 1:5,000), anti-FLAG-HRP (M2, Sigma, 1:5,000), anti-myc-HRP antibodies (9E10, Roche, 1:5,000), anti-His-HRP (Sigma, 1:2,000), anti-GST-HRP (Abcam, 1:10,000), mouse monoclonal anti-Ub (PAD1) (Santa Cruz Biotechnology, 1:2,000) and goat anti-mouse IgG-HRP (Santa Cruz, 1:10,000). Proteins were visualized using the Immobilon kit (Millipore) under standard conditions. Densitometry of proteins was calculated using the Image J software. Fluorimetric GUS assays Thirty-six hours after transient expression of proteins in N. benthamiana, plant tissue was ground in liquid nitrogen, homogenized in GUS buffer (50 mM NaPO4, pH 7; 10 mM β-mercaptoethanol; 10 mM NaEDTA; 0.1% Sarcosyl; 0.1% Triton X-100), and centrifuged for 5 min at 10,000 g . One microgram of total protein in supernatants was used to fluorimetrically measure enzymatic GUS activities using 4-methylumbelliferyl-β- D -glucuronide as substrate in a microtiter fluorimeter (FL600, Bio-Tek, Highland Park, VT, USA). Standard curves were prepared with a range of increasing concentrations of 4-methylumbelliferone (Sigma-Aldrich). Mean values and s.e.m. values were calculated from the results of eight independent experiments (2–4 replicates/experiment). Quantification of cell death using electrolyte leakage Four leaf discs (6 mm diameter) were harvested 24 hpi, washed and incubated at room temperature in 5 ml of distilled water before measuring conductivity. Four independent experiments were performed with three plants (four leaves per plant). RNA extraction and quantitative RT-PCR analysis Material for RNA analysis was ground in liquid nitrogen and total RNA was isolated using the Nucleospin RNA plant kit (Macherey-Nagel), according to the manufacturer’s recommendations. Reverse transcription was performed using 1.5 μg of total RNA. Quantitative RT-PCR (Q-RT-PCR) was performed on a Light Cycler 480 II machine (Roche Diagnostics, Meylan, France), using Roche reagents. Primers used for Q-RT-PCR are provided as Supplementary Information . Relative expression was calculated as the ΔCp between each gene and the average of internal controls ( SAND family (At2g28390) and β-tubulin 4 (At5g44340)). Average ΔCp was calculated from three experimental replicates and related to the value of each gene at time 0, which is set at 1. How to cite this article: Marino, D. et al . Arabidopsis ubiquitin ligase MIEL1 mediates degradation of the transcription factor MYB30 weakening plant defence. Nat. Commun. 4:1476 doi: 10.1038/ncomms2479 (2013).